Alendronate inhalation ameliorates elastase-induced pulmonary emphysema in mice by induction of apoptosis of alveolar macrophages Alveolar macrophages play a crucial role in the pathogenesis of emphysema, for which there is currently no effective treatment. Bisphosphonates are widely used to treat osteoclast-mediated bone diseases. Here we show that delivery of the nitrogen-containing bisphosphonate alendronate via aerosol inhalation ameliorates elastase-induced emphysema in mice. Inhaled, but not orally ingested, alendronate inhibits airspace enlargement after elastase instillation, and induces apoptosis of macrophages in bronchoalveolar fluid via caspase-3- and mevalonate-dependent pathways. Cytometric analysis indicates that the F4/80 + CD11b high CD11c mild population characterizing inflammatory macrophages, and the F4/80 + CD11b mild CD11c high population defining resident alveolar macrophages take up substantial amounts of the bisphosphonate imaging agent OsteoSense680 after aerosol inhalation. We further show that alendronate inhibits macrophage migratory and phagocytotic activities and blunts the inflammatory response of alveolar macrophages by inhibiting nuclear factor-κB signalling. Given that the alendronate inhalation effectively induces apoptosis in both recruited and resident alveolar macrophages, we suggest this strategy may have therapeutic potential for the treatment of emphysema. Chronic obstructive pulmonary disease (COPD) is characterized by airflow limitation, which is usually progressive and associated with chronic inflammatory and immune responses of the small airways [1] . COPD is associated with significant mortality. It also increases the risk of lung cancer [2] , causes disability and impairs the quality of life. Recent advances in the management of COPD have reduced the frequency and severity of exacerbations, and improved health status and exercise tolerance. COPD is a complex inflammatory disease involving many types of inflammatory cells, such as macrophages, neutrophils, B cells, lymphoid aggregates and CD4 + and CD8 + T cells [3] , [4] . Among these cell types, alveolar macrophages are important effector cells in COPD because of their production of a host of inflammatory mediators, including reactive oxygen species, cytokines, chemokines, growth factors and proteases [4] , [5] , [6] . Increasing severity of COPD is associated with increases in the number and elastinolytic activity of alveolar macrophages in the airway, lung parenchyma, bronchoalveolar lavage (BAL) fluid and sputum [7] , [8] , [9] . Moreover, alveolar macrophages are known to have prolonged survival in smokers with elevated macrophage levels of anti-apoptotic proteins [10] . However, few studies have demonstrated effective strategies for suppressing activated alveolar macrophages in COPD. Bisphosphonates are potent inhibitors of bone resorption and have been widely used in the treatment of metabolic bone diseases such as osteoporosis, Paget’s disease and metastatic bone disease [11] , [12] , [13] . Bisphosphonates are pyrophosphate analogues that contain a phosphate–carbon–phosphate (P–C–P) backbone. They mainly exert their effects on osteoclasts in vivo at the sites of active bone remodelling, particularly in areas undergoing osteoclastic resorption [14] , [15] . Most of the cell type-specific effects of bisphosphonates are a function of their P–C–P structure, which imparts a strong binding affinity for hydroxyapatite on bone mineral surfaces. Compared with ‘simple’ bisphosphonates (for example, etidronate and clodronate), nitrogen-containing bisphosphonates (for example, alendronate, risedronate and zoledronate) exert more potent antiresorptive effects. These nitrogen-containing bisphosphonates inhibit farnesyl pyrophosphate (FPP) synthase, a key enzyme in the mevalonate pathway, resulting in disrupted synthesis of the isoprenoid intermediates, FPP and geranylgeranyl pyrophosphate (GGPP), which are crucial for the correct subcellular localization and function of small GTP-binding proteins such as Rac and Ras [16] , [17] . Loss of isoprenylated proteins leads to osteoclast apoptosis. Bisphosphonates have been shown to induce apoptosis in macrophage cell lines such as RAW264 and J774 cells [18] , [19] , and pinocytotic activity of the monocyte/macrophage lineage has been suggested to contribute to the ability of these cells to take up sufficient amounts of bisphosphonates [20] . However, it remains to be determined whether alveolar macrophages are similarly affected by bisphosphonates. In this study, we investigated the effects of bisphosphonates on alveolar macrophages in an elastase-induced mouse model of COPD in vivo . We examined the effect of alendronate administration to the lung via aerosol inhalation on lung morphology and cellular indices of inflammation. We also determined the mechanisms of alendronate action in vitro in primary alveolar macrophages and MH-S mouse alveolar macrophages. To the best of our knowledge, this is the first study to demonstrate the effective suppression of alveolar macrophages via aerosol inhalation of alendronate. Aerosol inhalation of alendronate may thus represent a novel, effective, non-invasive and safe therapeutic treatment for alveolar macrophage-mediated lung diseases, including COPD. Effect of inhaled alendronate on elastase-induced emphysema We investigated the effects of aerosol inhalation of alendronate on COPD in a model of emphysema generated by intratracheal instillation of elastase. Elastase-induced acute lung injury is characterized by substantial infiltration of neutrophils and macrophages within 24 h, and by subsequent destruction of the alveolar wall and airspace enlargement, resembling human emphysema [21] . We evaluated the efficacy of bisphosphonates for ameliorating alveolar macrophage-mediated inflammation by examining the effects on lung pathology of alendronate, administered to the lung via aerosol inhalation, in this mouse emphysema model. Alendronate was administered at 0.33–3.25 μg per mouse, which was comparable to or less than the dose used for oral administration in humans (about 5 mg per day). Examination of BAL fluids in the elastase-induced mouse model revealed significant increases in the numbers of macrophages (major cell type), neutrophils and lymphocytes at day 1, and these remained elevated at day 7 ( Fig. 1a ). Airspaces were significantly enlarged, and the mean linear intercept was increased at day 7 with a further increase at day 21 ( Fig. 1b ). Alendronate inhalation (0.33–3.25 μg per mouse) on days 7 and 14 effectively inhibited airspace enlargement and reduced the mean linear intercept measured at 21 days after elastase instillation, whereas alendronate inhalation alone had no effect on lung morphology in control mice ( Fig. 2a ). The inhibitory effects of alendronate on elastase-induced alveolar enlargement were dose dependent from 0.33 to 3.25 μg ( Fig. 2b ). Inhalation of alendronate 3.25 μg on day 7 alone inhibited alveolar enlargement as effectively as inhalation of 3.25 μg on days 7 and day 14 ( Fig. 2c ). 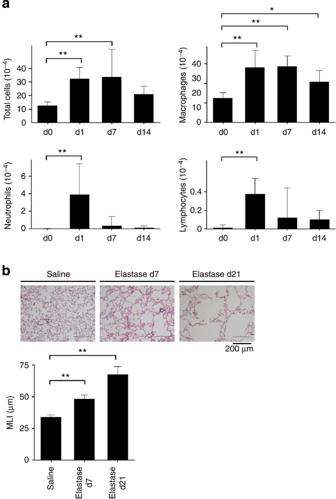Figure 1: Analysis of elastase-induced emphysema model mice. Elastase (15 μg per mouse) or saline was instilled into C57BL/6 mice intratracheally. BAL was performed on days 1, 7 and 14 (a). BAL total cell, macrophage, neutrophil and lymphocyte counts were made using a haemocytometer and hema-3-stained cytospins (n=5 mice per group). Lung sections at days 7 and 21 were stained with haematoxylin and eosin (b) (magnification, × 200). Scale bar, 200 μm. Semiquantitative analysis of lung tissue using mean linear intercept (MLI) is shown (n=5 mice per group). Data represent mean values±s.d. *P<0.05, **P<0.01 versus elastase administration at that point, measured by one-way analysis of variance with Tukey’spost hoctest. Figure 1: Analysis of elastase-induced emphysema model mice. Elastase (15 μg per mouse) or saline was instilled into C57BL/6 mice intratracheally. BAL was performed on days 1, 7 and 14 ( a ). BAL total cell, macrophage, neutrophil and lymphocyte counts were made using a haemocytometer and hema-3-stained cytospins ( n =5 mice per group). Lung sections at days 7 and 21 were stained with haematoxylin and eosin ( b ) (magnification, × 200). Scale bar, 200 μm. Semiquantitative analysis of lung tissue using mean linear intercept (MLI) is shown ( n =5 mice per group). Data represent mean values±s.d. * P <0.05, ** P <0.01 versus elastase administration at that point, measured by one-way analysis of variance with Tukey’s post hoc test. 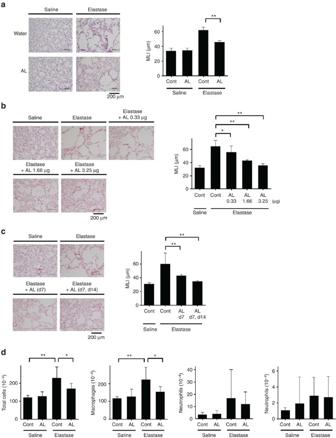Figure 2: Effect of inhaled alendronate on elastase-induced emphysema in mice. Elastase (15 μg per mouse) or saline was instilled into C57BL/6 mice intratracheally. The mice were then treated intratracheally with alendronate (AL; 3.25 μg per mouse) or water on days 7 and 14. Lung sections at day 21 were stained with haematoxylin and eosin (aleft; magnification, × 200). Scale bar, 200 μm. Semiquantitative analysis of lung tissue using mean linear intercept is shown (aright;n=15 mice per group). Data represent mean values±s.d. *P<0.05, **P<0.01 versus saline/elastase treated with water or alendronate, measured by one-way analysis of variance with Tukey’spost hoctest (a). Elastase-induced emphysema mice were treated intratracheally with alendronate (0.33, 1.66 or 3.25 μg per mouse) on days 7 and 14 (b) and with 3.25 μg per mouse on day 7 only, or on days 7 and 14 (c). Lung sections at day 21 were stained with haematoxylin and eosin (left; magnification, × 200). Scale bar, 200 μm. Semiquantitative analysis of lung tissue using mean linear intercept is shown (right;n=5 mice per group). BAL was performed on day 9 (d). BAL total cell, macrophage, neutrophil and lymphocyte counts were made using a haemocytometer and hema-3-stained cytospins (n=5 mice per group). Data represent mean values±s.d. *P<0.05, **P<0.01 versus control or elastase treated with alendronate at that dose (b) or that point (c), or saline/elastase treated with water or alendronate (d), measured by one-way analysis of variance with Tukey’spost hoctest (b–d). Full size image Figure 2: Effect of inhaled alendronate on elastase-induced emphysema in mice. Elastase (15 μg per mouse) or saline was instilled into C57BL/6 mice intratracheally. The mice were then treated intratracheally with alendronate (AL; 3.25 μg per mouse) or water on days 7 and 14. Lung sections at day 21 were stained with haematoxylin and eosin ( a left; magnification, × 200). Scale bar, 200 μm. Semiquantitative analysis of lung tissue using mean linear intercept is shown ( a right; n =15 mice per group). Data represent mean values±s.d. * P <0.05, ** P <0.01 versus saline/elastase treated with water or alendronate, measured by one-way analysis of variance with Tukey’s post hoc test ( a ). Elastase-induced emphysema mice were treated intratracheally with alendronate (0.33, 1.66 or 3.25 μg per mouse) on days 7 and 14 ( b ) and with 3.25 μg per mouse on day 7 only, or on days 7 and 14 ( c ). Lung sections at day 21 were stained with haematoxylin and eosin (left; magnification, × 200). Scale bar, 200 μm. Semiquantitative analysis of lung tissue using mean linear intercept is shown (right; n =5 mice per group). BAL was performed on day 9 ( d ). BAL total cell, macrophage, neutrophil and lymphocyte counts were made using a haemocytometer and hema-3-stained cytospins ( n =5 mice per group). Data represent mean values±s.d. * P <0.05, ** P <0.01 versus control or elastase treated with alendronate at that dose ( b ) or that point ( c ), or saline/elastase treated with water or alendronate ( d ), measured by one-way analysis of variance with Tukey’s post hoc test ( b – d ). Full size image We evaluated the effect of alendronate inhalation on the elastase-induced inflammatory response by counting the number of inflammatory cells in the BAL fluid. Alendronate inhalation 7 days after elastase instillation significantly decreased the total cell and macrophage counts, while neutrophil and lymphocyte counts in the BAL fluid were unaffected by alendronate inhalation ( Fig. 2d ). To determine if the effects of inhaled alendronate on elastase-induced emphysema were specific to alendronate, we repeated the experiments using risedronate, another nitrogen-containing bisphosphonate. As expected, 3.5 μg of risedronate significantly inhibited alveolar enlargement and elastase-induced macrophage accumulation in BAL fluids ( Supplementary Fig. 1a,b ). We also investigated the effects of inhaled alendronate on acute lung injury in mice challenged with intratracheal administration of Escherichia coli lipopolysaccharide (LPS). The numbers of macrophages in BAL fluid were slightly increased, but the numbers of neutrophils at day 3 and numbers of lymphocytes at day 7 were significantly increased ( Supplementary Fig. 2a ). Alendronate inhalation had no effects on numbers of neutrophils and lymphocytes in this model ( Supplementary Fig. 2b,c ). These results suggest that the effects of alendronate on lung injury depend on the injury model, and the beneficial effects of alendronate on elastase-induced emphysema are unlikely to be associated with nonspecific anti-inflammatory mechanisms, but are more likely to be caused by the inhibition of selective macrophage-mediated immunological and pathological processes. Effect of inhaled alendronate on smoking-induced emphysema We studied the effects of alendronate in a different emphysema model generated by whole-body exposure to cigarette smoke, as described previously [22] , [23] . This model was characterized by the infiltration of immune and inflammatory cells after 2 months, and by airspace enlargement after prolonged exposure (>6 months), similar to the response observed in humans. Alendronate inhalation effectively reduced the macrophage accumulation and emphysematous changes in this model ( Fig. 3a,b ). These data suggest that alendronate selectively inhibited airspace enlargement and the accumulation of alveolar macrophages in cigarette smoke-induced emphysema. 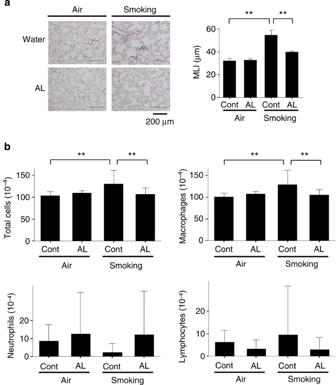Figure 3: Effect of inhaled alendronate on smoking-induced emphysema in mice. C57BL/6 mice were subjected to smoke from two unfiltered cigarettes per day, 6 days a week for 6 months. Alendronate (3.25 μg per mouse) was administered intratracheally at 1, 2, 3, 4 and 5 months after the start of smoking stimulation. Lung sections at 6 months were stained with haematoxylin and eosin (a) (left; magnification, × 200). Semiquantitative analysis of lung tissue using mean linear intercept is shown (right;n=5 mice per group). BAL was performed at 2 months (b). BAL total cell, macrophage, neutrophil and lymphocyte counts were performed using a haemocytometer and hema-3-stained cytospins (n=5 mice per group). Data represent mean values±±s.d. *P<0.05, **P<0.01 air/smoke treated with water or alendronate, measured by one-way analysis of variance with Tukey’spost hoctest (a,b). Figure 3: Effect of inhaled alendronate on smoking-induced emphysema in mice. C57BL/6 mice were subjected to smoke from two unfiltered cigarettes per day, 6 days a week for 6 months. Alendronate (3.25 μg per mouse) was administered intratracheally at 1, 2, 3, 4 and 5 months after the start of smoking stimulation. Lung sections at 6 months were stained with haematoxylin and eosin ( a ) (left; magnification, × 200). Semiquantitative analysis of lung tissue using mean linear intercept is shown (right; n =5 mice per group). BAL was performed at 2 months ( b ). BAL total cell, macrophage, neutrophil and lymphocyte counts were performed using a haemocytometer and hema-3-stained cytospins ( n =5 mice per group). Data represent mean values±±s.d. * P <0.05, ** P <0.01 air/smoke treated with water or alendronate, measured by one-way analysis of variance with Tukey’s post hoc test ( a , b ). Full size image In vivo lung uptake of inhaled bisphosphonates We visualized the uptake of the near-infrared bisphosphonate imaging agent OsteoSense680, administered via aerosol inhalation or intragastric injection (oral gavage), in mouse lung cells. Staining of freshly isolated lung tissue demonstrated signals from the inhaled OsteoSense680 probe primarily in elastase- but not saline-instilled lungs ( Fig. 4a ). Only low signals were detected in bone ( Fig. 5a–c ). We investigated the cell types that took up OsteoSense680 in control lungs by multilabel flow cytometry analysis using markers to distinguish among macrophages, dendritic cells, B cells, T cells and NK cells ( Fig. 4b ). Both CD11b high and CD11b low fractions took up OsteoSense680 similarly, while the F4/80 + CD11b high fraction contained Ly6C mild high inflammatory monocytic cells in saline-instilled lungs. Elastase instillation increased the F4/80 + CD11b high fraction from ∼ 44.2% (8.24% per 18.64%) to 53% (12.5% per 23.6%) ( Fig. 4c ), with a preferential increase in the Ly6C mild high CD301 low population. These data suggest that most of the CD11b high OsteoSense680 + cells exhibited surface characteristics of M1 macrophages. 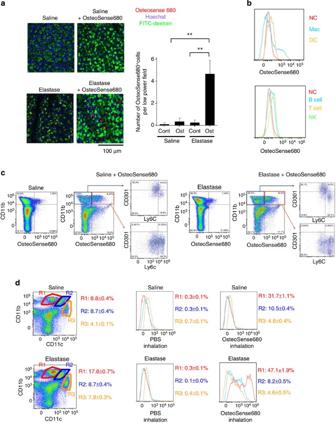Figure 4: Uptake of aerosol inhaled OsteoSense680 by alveolar macrophagesin vivo. C57BL/6 mice were treated with OsteoSense680 (Ost; 3.25 μg per mouse) or PBS intratracheally on day 7 after elastase or saline instillation. Lung tissues were examined at day 1 by fluorescence microscopy (a) (magnification, × 40;n=5 mice per group). Scale bar, 100 μm. Data represent mean values±s.d. *P<0.05, **P<0.01 versus saline/elastase treated with water or OsteoSense680, measured by one-way analysis of variance with Tukey’spost hoctest (a). Tissues were counterstained with FITC-dextran (vessels) and Hoechst 33342 (nuclei). The types of cells that took up OsteoSense680 were analysed by flow cytometry (b). Macrophages (F4/80+CD11b+), dendritic cells (CD11c+CD206+), B cells (CD19+CD22+), T cells (CD3+) and NK cells (CD3−CD94+) are shown. The types of macrophage (F4/80+CD11b+) affected by OsteoSense680 in elastase- and saline-instilled mice were further analysed for Ly6C and CD301 expression; M1 macrophages (CD11b+Ly6C+mild highCD301low) and M2 macrophages (CD11b+Ly6clowCD301mild high) (c) (n=5 mice per group). The subpopulations of lung macrophages (F4/80+) that took up OsteoSense68 in saline- and elastase-instilled lungs were determined. R1: CD11bhighCD11clowF4/80+; R2: CD11bhighCD11chighF4/80+; R3: CD11blowCD11chighF4/80+(d) (n=4 mice per group). Figure 4: Uptake of aerosol inhaled OsteoSense680 by alveolar macrophages in vivo. C57BL/6 mice were treated with OsteoSense680 (Ost; 3.25 μg per mouse) or PBS intratracheally on day 7 after elastase or saline instillation. Lung tissues were examined at day 1 by fluorescence microscopy ( a ) (magnification, × 40; n =5 mice per group). Scale bar, 100 μm. Data represent mean values±s.d. * P <0.05, ** P <0.01 versus saline/elastase treated with water or OsteoSense680, measured by one-way analysis of variance with Tukey’s post hoc test ( a ). Tissues were counterstained with FITC-dextran (vessels) and Hoechst 33342 (nuclei). The types of cells that took up OsteoSense680 were analysed by flow cytometry ( b ). Macrophages (F4/80 + CD11b + ), dendritic cells (CD11c + CD206 + ), B cells (CD19 + CD22 + ), T cells (CD3 + ) and NK cells (CD3 − CD94 + ) are shown. The types of macrophage (F4/80 + CD11b + ) affected by OsteoSense680 in elastase- and saline-instilled mice were further analysed for Ly6C and CD301 expression; M1 macrophages (CD11b + Ly6C +mild high CD301 low ) and M2 macrophages (CD11b + Ly6c low CD301 mild high ) ( c ) ( n =5 mice per group). The subpopulations of lung macrophages (F4/80 + ) that took up OsteoSense68 in saline- and elastase-instilled lungs were determined. R1: CD11b high CD11c low F4/80 + ; R2: CD11b high CD11c high F4/80 + ; R3: CD11b low CD11c high F4/80 + ( d ) ( n =4 mice per group). 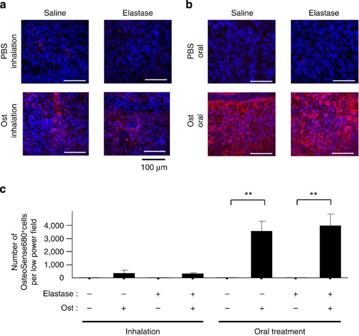Figure 5: Uptake of aerosol inhaled or oral OsteoSense680 in bone. C57BL/6 mice were treated with OsteoSense680 (3.25 μg per mouse) or PBS intratracheally on day 7 after elastase or saline instillation. Bone tissues on day 1 were examined by fluorescence microscopy (a–c) (magnification, × 40;n=4 mice per group). Scale bar, 100 μm. The tissues were counterstained with Hoechst 33342 (nucleus). Data represent mean values±s.d from triplicate experiments. *P<0.05, **P<0.01 versus saline/elastase treated with water or OsteoSense680 by inhaled or oral administration, measured by one-way analysis of variance with Tukey’spost hoctest (c). Full size image Figure 5: Uptake of aerosol inhaled or oral OsteoSense680 in bone. C57BL/6 mice were treated with OsteoSense680 (3.25 μg per mouse) or PBS intratracheally on day 7 after elastase or saline instillation. Bone tissues on day 1 were examined by fluorescence microscopy ( a – c ) (magnification, × 40; n =4 mice per group). Scale bar, 100 μm. The tissues were counterstained with Hoechst 33342 (nucleus). Data represent mean values±s.d from triplicate experiments. * P <0.05, ** P <0.01 versus saline/elastase treated with water or OsteoSense680 by inhaled or oral administration, measured by one-way analysis of variance with Tukey’s post hoc test ( c ). Full size image We further characterized the macrophage subpopulations that were increased by elastase instillation in cells isolated from lungs and separated by flow cytometry using CD11b and CD11c antibodies. Three clustered cell subpopulations (gated as R1–R3) were identified. The R1-gated region contained CD11b high CD11c low cells, the R2-gated region CD11b high Cd11c high cells and the R3-gated region CD11b low CD11c high cells. The R1- and R3-gated populations were significantly increased in response to elastase instillation compared with saline instillation (17.8±0.7 versus 8.8±0.4%, 7.8±0.3 versus 4.1±0.1%; P <0.05; Fig. 4d ), while the R2-gated populations were similar in saline-and elastase-instilled lungs (8.7±0.4 versus 8.7±0.4%; Fig. 4d ). In addition, the R1-gated population took up most OseoSense680 in both saline- and elastase-instilled lungs (47.1±1.9 versus 31.7±1.1%; Fig. 4d and Supplementary Table 2b ). These data indicate that F4/80 + CD11b high CD11c low alveolar macrophages were mainly responsible for bisphosphonate uptake in an elastase-induced emphysema model, though the R3-gated population also took up bisphosphonates to a lesser extent. To determine the extrapulmonary distribution of bisphosphonates delivered via inhalation or oral gavage, OsteoSense680 was examined in bone, bone marrow, spleen and peripheral blood. In addition to the lung, week-inhaled OsteoSense680 accumulation was detected in bone, with low or absent levels in bone marrow and spleen in saline-instilled mice, and no measurable increases in signals in elastase-instilled mice ( Supplementary Table 1 ). Induction of macrophage apoptosis by alendronate in vivo Apoptosis of alveolar macrophages in elastase-instilled lungs was examined by immunofluorescence. Alendronate inhalation 7 days after elastase instillation markedly increased TUNEL (terminal deoxynucleotidyl transferase-mediated dUTP nick end labelling)- and F40/80-positive cells at day 21, assessed by double immunofluorescence ( Fig. 6a,b ). These results indicate that alendronate inhalation reduced the accumulation of alveolar macrophages, at least partly, by inducing apoptosis of those cells in vivo . 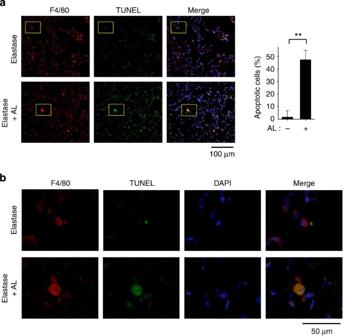Figure 6: Induction of macrophage apoptosis by aerosol inhaled alendronate in elastase-induced emphysemain vivo. C57BL/6 mice were treated with alendronate (3.25 μg per mouse) or water intratracheally on day 7 after elastase (15 μg per mouse;n=5 mice per group). Lung tissues at day 2 were subjected to immunofluorescence staining to determine the co-localization of alveolar macrophages (F4/80 stain; red), apoptotic cells (TUNEL stain; green) and nucleus (4′,6-diamino-2-phenylindole (DAPI); blue) (a) (magnification, × 200) and (b) (magnified view of the area outlined with a yellow square). Scale bar, 100 μm (a), 50 μm (b). Data represent mean values±s.d. *P<0.05, **P<0.01 versus elastase treated with water or alendronate, measured by Student’st-test (a). Figure 6: Induction of macrophage apoptosis by aerosol inhaled alendronate in elastase-induced emphysema in vivo. C57BL/6 mice were treated with alendronate (3.25 μg per mouse) or water intratracheally on day 7 after elastase (15 μg per mouse; n =5 mice per group). Lung tissues at day 2 were subjected to immunofluorescence staining to determine the co-localization of alveolar macrophages (F4/80 stain; red), apoptotic cells (TUNEL stain; green) and nucleus (4′,6-diamino-2-phenylindole (DAPI); blue) ( a ) (magnification, × 200) and ( b ) (magnified view of the area outlined with a yellow square). Scale bar, 100 μm ( a ), 50 μm ( b ). Data represent mean values±s.d. * P <0.05, ** P <0.01 versus elastase treated with water or alendronate, measured by Student’s t -test ( a ). Full size image Effect of oral alendronate on elastase-induced emphysema We examined the effects of oral administration of alendronate on elastase-induced morphological changes in the lung. Alendronate administered by oral gavage on days 7 and 14 after elastase instillation failed to inhibit airspace enlargement and did not reduce the mean linear intercept measured at 21 days after elastase instillation ( Fig. 7a ). These results were consistent regardless of the alendronate dosage and number of administrations ( Fig. 7b,c ). 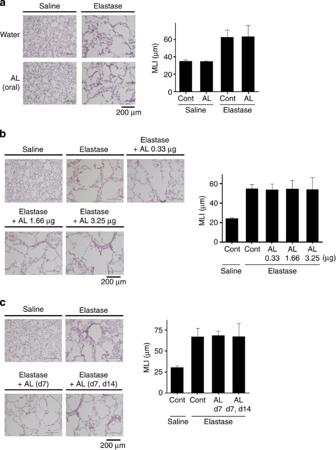Figure 7: Effect of oral administration of alendronate on elastase-induced emphysema in mice. Elastase (15 μg per mouse) or saline was instilled into C57BL/6 mice intratracheally, followed by oral alendronate (3.25 μg per mouse) or water on days 7 and 14. Lung sections at day 21 were stained with haematoxylin and eosin (aleft; magnification, × 200). Scale bar, 200 μm. Semiquantitative analysis of lung tissue using mean linear intercept is shown (aright;n=15 mice per group). Data represent mean values±s.d. *P<0.05, **P<0.01 versus saline/elastase treated with water or alendronate, measured by one-way analysis of variance with Tukey’spost hoctest (a). Elastase-induced emphysema mice were treated with oral alendronate at 0.33, 1.66 or 3.25 μg per mouse) on days 7 and 14 (b) and with 3.25 μg per mouse on day 7 only, or on days 7 and 14 (c). Lung sections at day 21 were stained with haematoxylin and eosin (left; magnification, × 200). Scale bar, 200 μm. Semiquantitative analysis of lung tissue using mean linear intercept is shown (right;n=5 mice per group). Data represent mean values±s.d. *P<0.05, **P<0.01 versus control or elastase treated with alendronate at that dose (b) or that point (c), measured by one-way analysis of variance with Tukey’spost hoctest (b,c). Figure 7: Effect of oral administration of alendronate on elastase-induced emphysema in mice. Elastase (15 μg per mouse) or saline was instilled into C57BL/6 mice intratracheally, followed by oral alendronate (3.25 μg per mouse) or water on days 7 and 14. Lung sections at day 21 were stained with haematoxylin and eosin ( a left; magnification, × 200). Scale bar, 200 μm. Semiquantitative analysis of lung tissue using mean linear intercept is shown ( a right; n =15 mice per group). Data represent mean values±s.d. * P <0.05, ** P <0.01 versus saline/elastase treated with water or alendronate, measured by one-way analysis of variance with Tukey’s post hoc test ( a ). Elastase-induced emphysema mice were treated with oral alendronate at 0.33, 1.66 or 3.25 μg per mouse) on days 7 and 14 ( b ) and with 3.25 μg per mouse on day 7 only, or on days 7 and 14 ( c ). Lung sections at day 21 were stained with haematoxylin and eosin (left; magnification, × 200). Scale bar, 200 μm. Semiquantitative analysis of lung tissue using mean linear intercept is shown (right; n =5 mice per group). Data represent mean values±s.d. * P <0.05, ** P <0.01 versus control or elastase treated with alendronate at that dose ( b ) or that point ( c ), measured by one-way analysis of variance with Tukey’s post hoc test ( b , c ). Full size image We also examined the distribution of orally delivered OsteoSense680. As expected, OsteoSense680 accumulated in the bone ( Fig. 5a–c ), but modest signals were also detected in saline-instilled lungs and were increased in elastase-instilled lungs (8.1±0.8 versus 1.4±0.2%; Supplementary Table 3 ). These data suggest that alendronate delivered via oral gavage would accumulate almost exclusively in bone, and would thus have little or no effect on the development of emphysema, although a little alendronate uptake was observed in lung macrophages. Induction of macrophage apoptosis by alendronate in vitro Bisphosphonates are known to inhibit bone resorption by inducing osteoclast apoptosis. Moreover, earlier studies showed that bisphosphonates induced apoptosis in other cell types, including macrophages (RAW264, J774A) and myeloid cells, which are derived from the monocyte lineage [18] , [19] . We therefore determined alendronate-induced apoptosis in alveolar macrophages. Alendronate increased caspase-3 levels in primary alveolar macrophages at 48 and 72 h in a dose-dependent manner ( Fig. 8a ). We also examined caspase-3 protein levels in MH-S cells, a cell line derived from mouse alveolar macrophages, by western blotting, because the protein yield from primary alveolar macrophages was very low. Cleaved caspase-3 protein levels were increased at 48 and 72 h after alendronate treatment (100 μM) in MH-S cells ( Fig. 8b ). 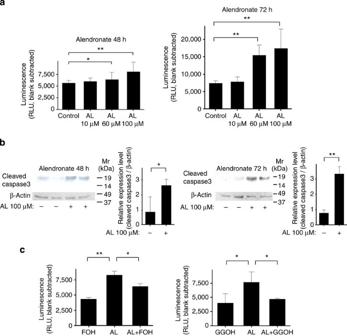Figure 8: Effect of alendronate on apoptosis of alveolar macrophagesin vitro. Primary alveolar macrophages were treated for 48 or 72 h with alendronate (10, 60, 100 μM), and apoptosis was analysed by caspase-3/7 assay (a). MH-S cells were treated for 48 or 72 h with alendronate (100 μM). Cells were harvested for the analysis of cleaved caspase-3 protein by western blotting (b). Primary alveolar macrophages were pretreated with FOH or GGOH followed by treatment for 48 h with alendronate (100 μM) (c). Apoptosis of macrophages was analysed by caspase-3/7 assay. Data represent mean values±s.d from triplicate experiments. *P<0.05, **P<0.01 versus control or alendronate group (a,b), or FOH or GGOH treated with alendronate (c), measured by one-way analysis of variance with Tukey’spost hoctest (a,c) or Student’st-test (b). Figure 8: Effect of alendronate on apoptosis of alveolar macrophages in vitro. Primary alveolar macrophages were treated for 48 or 72 h with alendronate (10, 60, 100 μM), and apoptosis was analysed by caspase-3/7 assay ( a ). MH-S cells were treated for 48 or 72 h with alendronate (100 μM). Cells were harvested for the analysis of cleaved caspase-3 protein by western blotting ( b ). Primary alveolar macrophages were pretreated with FOH or GGOH followed by treatment for 48 h with alendronate (100 μM) ( c ). Apoptosis of macrophages was analysed by caspase-3/7 assay. Data represent mean values±s.d from triplicate experiments. * P <0.05, ** P <0.01 versus control or alendronate group ( a , b ), or FOH or GGOH treated with alendronate ( c ), measured by one-way analysis of variance with Tukey’s post hoc test ( a , c ) or Student’s t -test ( b ). Full size image Effect of FPP and GGPP on apoptosis by alendronate Nitrogen-containing bisphosphonates, including alendronate, induce apoptosis in osteoclasts by inhibiting enzymes of the mevalonate pathway, resulting in the loss of isoprenoid intermediates such as FPP and GGPP required for post-translational modification of small GTP-binding proteins (isoprenylation) [16] . We investigated the inhibition of protein isoprenylation in alendronate-induced apoptosis of alveolar macrophages by examining the effects of 50 μM farnesol (FOH) and 50 μM geranylgeraniol (GGOH), cell-permeable analogues of FPP and GGPP, respectively, on alendronate-induced apoptosis. Alendronate-induced apoptosis in primary alveolar macrophages was effectively abolished by FOH and GGOH at 48 and 72 h ( Fig. 8c ). Moreover, 50 μM FOH and 50 μM GGOH clearly prevented the alendronate-induced loss of viability of alveolar macrophages (data not shown). These results indicate that alendronate-induced apoptosis and reduced cellular viability were caused via the inhibition of mevalonate pathways in alveolar macrophages. Effects of alendronate on the function of alveolar macrophages We examined the effects of alendronate on the viability of alveolar macrophages by 3-(4,5-dimethylthiazol-2-yl)-2.5-diphenyl-2H-tetrazolium (MTT) assay. Alendronate reduced the viability of cultured primary alveolar macrophages at 48 and 72 h, in a dose-dependent manner ( Fig. 9a ). Moreover, alendronate treatment suppressed phagocytosis (fluorescein isothiocyanate (FITC)-dextran uptake) and migration (transwell migration) of cultured primary alveolar macrophages treated with 100 μM alendronate at 48 h ( Fig. 9b,c ). These results suggest that alendronate also reduced the activity of alveolar macrophages. 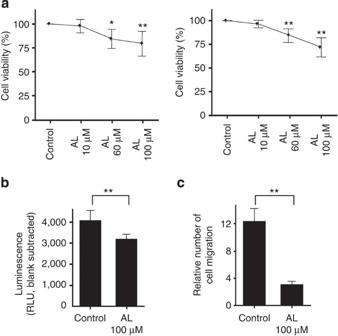Figure 9: Effects of alendronate on viability, phagocytosis capability and migration of alveolar macrophagesin vitro. Primary alveolar macrophages were treated for 48 or 72 h with alendronate (10, 60, 100 μM) and their viability was analysed by MTT assay (a). Alveolar macrophages treated with alendronate were incubated with FITC-dextran and phagocytosis was analysed by FITC-dextran uptake (b). Migration of alveolar macrophages treated with alendronate into 5-μm pore size polycarbonate membranes was measured by chemotaxis assay (c). Data represent mean values±s.d. from triplicate experiments. *P<0.05, **P<0.01 versus control or alendronate group (a–c), measured by one-way analysis of variance with Tukey’spost hoctest (a) or Student’st-test (b,c). Figure 9: Effects of alendronate on viability, phagocytosis capability and migration of alveolar macrophages in vitro. Primary alveolar macrophages were treated for 48 or 72 h with alendronate (10, 60, 100 μM) and their viability was analysed by MTT assay ( a ). Alveolar macrophages treated with alendronate were incubated with FITC-dextran and phagocytosis was analysed by FITC-dextran uptake ( b ). Migration of alveolar macrophages treated with alendronate into 5-μm pore size polycarbonate membranes was measured by chemotaxis assay ( c ). Data represent mean values±s.d. from triplicate experiments. * P <0.05, ** P <0.01 versus control or alendronate group ( a – c ), measured by one-way analysis of variance with Tukey’s post hoc test ( a ) or Student’s t -test ( b , c ). Full size image Inflammatory response of alveolar macrophages by alendronate We verified the anti-inflammatory and anti-proteinase effects of alendronate in alveolar macrophages in vitro by measuring the production of inflammatory cytokines and matrix metalloproteinase (MMP) after LPS stimulation (100 ng ml −1 ) in the presence of alendronate (100 μM) in MH-S cells. Pretreatment of MH-S cells with alendronate for 48 h attenuated phospho-nuclear factor (NF)-κB protein production following LPS stimulation for 30 min, while total NF-κB levels were unchanged, as evaluated by western blot analysis ( Fig. 10a ). Consistent with these results, 4-h LPS-induced increases in tumour necrosis factor (TNF)-α, interleukin (IL)-1β, IL-6 and monocyte chemoattractant protein (MCP)-1 protein levels were significantly blunted by prior treatment with alendronate for 48 h ( Fig. 10b ). Moreover, the induction of MMP-9 protein following LPS treatment for 24 h was reduced by prior treatment with alendronate for 48 h ( Fig. 10c ). These data indicate that alendronate suppressed the production of proinflammatory cytokines and MMP-9 via the inhibition of NF-κB signalling in alveolar macrophages. 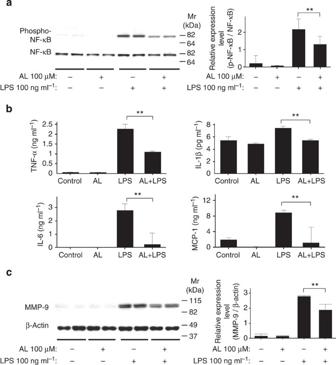Figure 10: Effect of alendronate on inflammatory response of alveolar macrophagein vitro. MH-S cells were treated for 48 h with alendronate (100 μM) and then stimulated with LPS (100 ng ml−1) for 30 min. Cells were then harvested for analysis of phospho-NF-κB and NF-κB by western blotting (aleft). Protein levels of phospho-NF-κB were normalized against protein levels of NF-κB (aright). Data represent mean values±s.d. from triplicate experiments. *P<0.05, **P<0.01 versus control or alendronate group, measured by one-way analysis of variance (ANOVA) with Tukey’spost hoctest (a). After 48 h of alendronate treatment and 4 h of LPS, culture media were analysed for TNF-α and IL-1β by ELISA and IL-6 and MCP-1 by cytometry bead array (b). After treatment with alendronate (100 μM) for 48 h and LPS (100 ng ml−1) for 24 h, the cells were harvested for analysis of MMP-9 by western blotting (cleft). Protein levels of MMP-9 were normalized against protein levels of β-actin (cright). Data represent mean values±s.d. from triplicate experiments. *P<0.05, **P<0.01 versus control or alendronate group, measured by one-way ANOVA with Tukey’spost hoctest (c). Figure 10: Effect of alendronate on inflammatory response of alveolar macrophage in vitro. MH-S cells were treated for 48 h with alendronate (100 μM) and then stimulated with LPS (100 ng ml −1 ) for 30 min. Cells were then harvested for analysis of phospho-NF-κB and NF-κB by western blotting ( a left). Protein levels of phospho-NF-κB were normalized against protein levels of NF-κB ( a right). Data represent mean values±s.d. from triplicate experiments. * P <0.05, ** P <0.01 versus control or alendronate group, measured by one-way analysis of variance (ANOVA) with Tukey’s post hoc test ( a ). After 48 h of alendronate treatment and 4 h of LPS, culture media were analysed for TNF-α and IL-1β by ELISA and IL-6 and MCP-1 by cytometry bead array ( b ). After treatment with alendronate (100 μM) for 48 h and LPS (100 ng ml −1 ) for 24 h, the cells were harvested for analysis of MMP-9 by western blotting ( c left). Protein levels of MMP-9 were normalized against protein levels of β-actin ( c right). Data represent mean values±s.d. from triplicate experiments. * P <0.05, ** P <0.01 versus control or alendronate group, measured by one-way ANOVA with Tukey’s post hoc test ( c ). Full size image Effects of phosphate on macrophage apoptosis by alendronate We determined if alendronate-induced apoptosis was affected by inorganic phosphate and dipalmitoyl phosphatidylcholine (DPPC), which are the most abundant single components of lung surfactant. Treatment of primary alveolar macrophages with 3 mM of inorganic phosphate alone had no effect on caspase-3/7 activities, but significantly enhanced alendronate-induced caspase-3/7 activities, measured by analysis of luminogenic substrate. DPPC alone increased caspase-3/7 activities but failed to increase their activities ( Supplementary Fig. 3a,b ) further in culture medium. These data indicate that the effects of alendronate on alveolar macrophages are dependent on the concentration of inorganic phosphate. Alveolar macrophages are known to act as critical effectors inducing inflammation and destruction of the alveolar wall and lung parenchyma in emphysema; however, no significant strategies specifically targeting these cells have yet been developed. In this study, we demonstrated that the delivery of alendronate via aerosol inhalation selectively induced apoptosis in alveolar macrophages and prevented airspace enlargement in elastase-induced emphysema in mice. Alendronate induced caspase-3-dependent apoptosis in alveolar macrophages and impaired cell viability, phagocytosis and migration in vitro , by inhibiting the mevalonate pathway. Alendronate also reduced LPS-induced production of inflammatory cytokines, such as TNF-α, IL-1β, IL-6 and MCP-1 via the inhibition of NF-κB signalling pathway, and MMPs such as MMP-9, from alveolar macrophages. Importantly, alendronate delivery via aerosol was capable of inducing apoptosis in alveolar macrophages. Earlier studies showed that macrophages, as well as osteoclasts, took up bisphosphonates by phagocytosis, and a liposome-encapsulated form of bisphosphonates induced macrophage depletion in organs and tissues in vivo [24] . However, the ability of bisphosphonates in a non-encapsulated form to suppress macrophage-mediated inflammatory responses in vivo remains to be investigated. The porcine pancreatic elastase-induced emphysema model [25] has been used for 40 years and represents a simple and reproducible model of emphysema that recapitulates some of the important pathological findings of human emphysema. Histologic examination showed that the alveolar wall was rapidly destroyed and many elastic fibres had disappeared by 24 h after elastase instillation [26] . Macrophages and neutrophils subsequently accumulated in the alveolar spaces resulting in progressive airspace enlargement over the first month following elastase instillation [27] . However, few studies using the elastase-induced emphysema model have investigated the abilities of agents administered after elastase instillation to protect the injured lung from structural alterations. In our study, alendronate was administered on day 7 after elastase instillation when the inflammatory response had already been robustly induced and on day 14. Our results also demonstrated a beneficial effect of alendronate inhalation on cigarette smoke-induced emphysema in mice. Alendronate, thus, effectively inhibited the progression of the inflammatory responses induced by elastase instillation and cigarette smoke, thereby demonstrating the potential therapeutic effect of alendronate inhalation for established emphysema. This evidence indicating that targeting of alveolar macrophages protects against elastase-induced emphysema suggests a potential therapeutic approach for the treatment of human emphysema, in which cigarette smoke is a major aetiologic factor. Although the main source of elastinolytic activity in the lungs of smokers remains controversial, alveolar macrophages, rather than neutrophils, have been suggested to play a critical role in the initiation and progression of emphysema in smokers, as well as in cigarette smoke-exposed animals [28] , [29] , [30] . Further studies are needed to evaluate the applicability of our findings to the clinical treatment of patients with COPD. Alendronate 100 μM significantly induced apoptosis in primary cultures of alveolar macrophages and in established MH-S cells, though this concentration is much higher than plasma concentrations (<0.25–0.34 μM) in humans administered therapeutic doses of 5–10 mg per day or 70 mg per week [31] . However, the alendronate dose administered to mice via aerosol inhalation was 3.25 μg, which was comparable to that used orally for the treatment of human bone diseases ( ∼ 5 mg per 50 kg). Given that the bioavailability of alendronate after oral intake is only 0.64%, skeletal uptake reaches 90% of the peak value within 1 h of oral administration, and alendronate disappears rapidly (0.5–2 h after oral administration) from the circulation [32] , the concentration in airways is likely to be negligible after oral administration. In contrast, the intratracheal administration of alendronate dry powder resulted in a 3.5-fold increase in bioavailability compared with oral treatment [33] . Flow cytometric analysis demonstrated that macrophages expressing both F4/80 and CD11b took up OsteoSense680 in response to elastase instillation, suggesting that Lys6C mild high CD301 low inflammatory macrophages or M1 macrophages undergo apoptosis in alendronate-treated lungs. F4/80 + CD11b high CD11c mild population is characterized inflammatory macrophages, and F4/80 + CD11b mild CD11c high population is defined resident alveolar macrophages. It was also notable that resident alveolar macrophages defined as F4/80 + CD11b low CD11c high were increased in elastase-instilled lungs and took up the OsteoSense680 probe. These results suggest that the inhalation of alendronate blocked the progression of emphysema via the suppression of pathogenic pathways mediated by inflammatory macrophages containing M1 macrophages, as well as resident alveolar macrophages. However, despite recent progress in our understanding of the differentiation of resident alveolar macrophages, interstitial macrophages and circulating monocytes, the recruitment process of alveolar macrophages remains unclear [34] . Our flow cytometric analysis demonstrated that aerosol instillation effectively targeted bisphosphonates to lung macrophages. Although technical parameters such as flow rate and aerosol particle size may affect the deposition of the drug in the lung, the results of this study demonstrate that intratracheal delivery of alendronate via aerosol is effective and feasible for the treatment of alveolar macrophage-mediated lung disease. The mechanisms whereby physiologically relevant doses of inhaled alendronate induce apoptosis in alveolar macrophages in vivo but not in vitro remain to be clarified. There are at least two possibilities, which are not mutually exclusive. First, resident alveolar macrophages in vivo may be activated by intratracheal elastase challenge, and activated alveolar macrophages are more likely to be able to internalize alendronate via pinocytosis, compared with non-activated macrophages. Indeed, alendronate inhalation had little or no effect on macrophage counts in control mice. Moreover, increased numbers of alveolar macrophages took up the bisphosphonate probe OsteoSense680 in elastase- but not saline-instilled lungs, as evaluated by fluorescent imaging and flow cytometry analyses. These results suggest that alveolar macrophages are capable of performing phagocytosis of non-encapsulated bisphosphonate in the inflammatory lung in vivo . Another possible explanation for the induction of alveolar macrophage apoptosis by low-dose bisphosphonate in vivo is that the alveolar space may serve as a unique environment where calcium phosphate is precipitated and bisphosphonate can bind to those precipitates with high affinity via its P–C–P backbone structure [35] . Alveolar type II epithelial cells produce and secrete pulmonary surfactant, a phospholipid-rich material lining the inside of the alveolar cells, and old surfactant is cleared from the alveolar space by alveolar type II epithelial cells and alveolar macrophages for degradation [36] . Inorganic phosphate released from the degraded phospholipids is transported from the alveolar space by the type IIb sodium–phosphate cotransporter, which is primarily expressed in alveolar type II epithelial cells [37] . This metabolism of pulmonary surfactant and inorganic phosphate in the alveolar space suggests that calcium phosphate may be more likely to be precipitated under conditions of alveolar type II epithelial cell damage, and calcium phosphate precipitate is bound by alendronate and then efficiently phagocytosed by alveolar macrophages. Indeed, 3-mM inorganic phosphate facilitated alendronate-induced apoptosis in cultured alveolar macrophages, whereas DPPC, a major phospholipid-forming surfactant particle, had no effect. In conclusion, the results of this study demonstrate that the inhalational administration of a clinically relevant dose of bisphosphonate can selectively reduce M1 macrophages and suppress alveolar airspace enlargement in an elastase-induced emphysema mouse model. Alendronate induces apoptosis in a caspase-3-dependent manner through inhibition of the mevalonate pathway in vitro . Alendronate can also suppress cell viability, phagocytosis and migration and the production of inflammatory cytokines and MMPs in alveolar macrophages. The non-invasiveness and feasibility of inhalational alendronate delivery may thus have important implications for the future treatment of COPD in which alveolar macrophages play a key pathogenic role. Antibodies and chemicals The following reagents were used: F4/80 (Santa Cruz Biotechnology, Santa Cruz, CA, USA), caspase-3, cleaved caspase-3, NF-κB, phospho-NF-κB (Cell Signaling Technology Inc., Danvers, MA, USA) and MMP-9 (Abcam, Cambridge, UK). Alendronate was provided by Merck & Co. Inc. (Whitehouse Station, NJ, USA). Mice All animal experiments were performed according to the guidelines of the Committee of Experimental Animal Research of Gunma University. For elastase-induced emphysema model mice, male 8-week-old C57BL/6 mice were anaesthetized and instilled with elastase (15 μg per mouse) intratracheally as an aerosol, using a microsprayer (Penn-Century Inc., Philadelphia, PA, USA). Control mice received saline. Alendronate (0.33–3.25 μg per mouse) was administered orally or intratracheally on days 7 and 14 after elastase instillation. Risedronate (3.5 μg per mouse; LKT Laboratories Inc., St Paul, MN, USA), another nitrogen-containing bisphosphonate, was administered intratracheally on days 7 and 14 after elastase instillation. These mice were killed at day 21 after elastase instillation for histological analysis. Smoking-induced emphysema was induced in female 8-week-old C57BL/6 mice by exposure to the smoke of two unfiltered cigarettes per day (University of Kentucky), 6 days a week for 6 months, using an experimental-smoking apparatus, as described previously [22] , [23] . Mice tolerated cigarette smoke exposure without evidence of toxicity (carboxyhaemoglobin levels about 10%). Alendronate (3.25 μg per mouse) was administered intratracheally at 1, 2, 3, 4 and 5 months after the start of cigarette smoking. These mice were killed at 2 months for BAL fluid analysis, and at 6 months for histological analysis. For the LPS-induced inflammatory model, male 8-week-old C57BL/6 mice were anaesthetized and instilled with LPS (1 mg kg −1 ; Sigma, St Louis, MO, USA) intratracheally as an aerosol using a microsprayer (Penn-Century Inc.). Control mice received saline. Alendronate (3.25 μg per mouse) was administered intratracheally on day 2 or 6 after LPS instillation. These mice were killed at 3 or 7 days after LPS instillation for BAL fluid analysis. Tissue processing Right lungs were inflated by instilling with 10% formalin at a constant pressure of 25-cm formalin (for 10 min) and fixed for 24 h before paraffin embedding. Serial sections were prepared for histological analysis. Bronchoalveolar lavage BAL was performed using a 20 G intravenous catheter inserted into the trachea. Lungs were lavaged four times with 0.75 ml PBS and then centrifuged at 1,000 g for 3 min. Cell pellets were resuspended in 1.0 ml PBS and used to determine total and differential cell counts using a haemocytometer and cytospins stained with a Diff-Quick stain kit (Sysmex, Kobe, Japan). Immunofluorescence Immunofluorescence labelling of lung sections was carried out using an antibody against F4/80 (1:100). Secondary antibodies were used for F4/80 staining an Alexa Fluor 488-conjugated mouse anti-rat IgG (1:100; Invitrogen Life Technologies Corp., Carlsbad, CA, USA). TUNEL staining was performed using the In situ Cell Death Detection Kit, Fluorescein (Roche, Mannheim, Germany) according to the manufacturer’s protocol. Lung tissue imaging Bisphosphonate distribution in living lungs was visualized by in vivo confocal microscopy, by modification of conventional methods [38] . Cy5-labelled bisphosphonate (OsteoSense680, Perkin Elmer Life Science, Boston, MA, USA) was administered to mice 24 h before the experiments. Fluorescein dextran (25 mg kg −1 body weight; Sigma) and Hoechst 33342 (10 mg kg −1 ; H1399, Invitrogen) were injected into the mice to visualize vessels and nuclei. Mice were killed and the lungs were removed. Living lung tissue was examined using a Nikon A1R system. The tissue was excited at wavelengths of 405, 561 and 640 nm. A × 40 (NA 1.15) water immersion objective lens (Nikon, Tokyo, Japan) was used, and the images were captured at 1.5 × zoom. More than five animals were examined in each group. Images were analysed using NIS-Elements software (Nikon). Preparations of cells and flow cytometry Stromal lung cells were isolated as described previously [39] , with minor modifications. In brief, mice were killed under general anaesthesia following systemic heparinization and lung tissues were collected. After removing the attached organs (heart, vessels, thymus) under a microscope, the tissue was cut into small pieces ( ∼ 1 mm 3 ) and centrifuged at 100 g for 4 min. The floating pieces were separated from the precipitate, which contained the blood cells, and incubated for 20 min in collagenase solution (2 mg ml −1 collagenase type 2 (Worthington) in Tyrode buffer) with gentle stirring. The digested tissue was centrifuged and the resultant pellet containing the SV fraction in PBS was resuspended and filtered through a 70-μm mesh. The dissociated SV cells were washed twice with PBS, incubated for 10 min in erythrocyte-lysing buffer as described previously [38] and finally resuspended in PBS supplemented with 3% fetal bovine serum. FcBlock antibody (553141, BD Pharmingen) was added at 60 ng per 1 × 10 6 cells followed by incubation on ice for 15 min. The isolated cells were incubated with either a labelled monoclonal antibody or isotype-matched control antibody and analysed by flow cytometry using a Canto II flow cytometer (BD Biosciences, San Diego, CA, USA) and FlowJo 7.2.2. software (Tomy Digital Biology). Dead cells were excluded by staining with propidium iodide (Invitrogen). The antibodies used were: anti-CD3 (145-2C11, BD Pharmingen), CD4 (RM4-5, BD Pharmingen), CD8a (53-6.7, BD Pharmingen), CD11b (M1/70, eBioscience, San Diego, CA, USA), CD11c (HL-3, eBioscience), CD19 (MB19-1, eBioscience), CD22.2 (CY34.1 BD Pharmingen, 2D6 Abcam, OX-97 Biolegend, San Diego, CA, USA), CD45R (RA3-6B2, Biolegend), CD94 (18d3, Biolegend), CD206 (MR5D3, Biolegend), CD244.2 (244F4, eBioscience), CD301 (ER-MP23, Serotec, Kidlington, UK), F4/80 (BM8, Caltag, Carlsbad, CA, USA), Ly6C (HK1.4, Biolegend) and NK1-1 (PK136, Biolegend). The OsteoSense680 signal was analysed using a band-pass filter for APC-Cy7 (excitation 633 nm and emission 780/60 nm). This set protocol was confirmed to isolate OsteoSense680 signals from other fluorochromes by preliminary experiments. Cell culture and stimulation Primary alveolar macrophages were collected from C57BL/6 mice by the BAL method. MH-S cells (derived from mouse alveolar macrophages) were obtained from ATCC. Cells were cultured in RPMI 1640 medium supplemented with 10% fetal bovine serum and 1% penicillin–streptomycin (Gibco Brl, Gaithersburg, MD, USA) at 37 °C in a 5% CO 2 atmosphere. Alendronate was added to the medium and the cells were incubated at 37 °C for 48 or 72 h. To examine the dependence on phosphoric acid and DPPC, a mixed solution of Na 2 HPO 4 and NaH 2 PO 4 (pH 7.4) was added to RPMI 1640 to a final concentration of 3.0 mM and 250 mg ml −1 DPPC (Sigma) was added. Alternatively, the cells were pretreated with FOH 50 μM (LKT Laboratories Inc., St Paul, MN, USA) or GGOH 50 μM (LKT) before alendronate administration. For the analysis of inflammation and protease production, LPS 100 ng ml −1 was added to the cells for 4 or 24 h after alendronate treatment. Caspase-3/7 assay Apoptosis in alveolar macrophages was investigated by measuring caspase-3/7 activities using Caspase-Glo 3/7 (Promega, Madison, MI, USA) according to the manufacturer’s protocol. This technique involved a luminogenic substrate containing the DEVD tetrapeptide. Luminescence was measured by ARVO HTS (Perkin Elmer). Cell viability assay The viability of alveolar macrophages was investigated by measuring cell viability using the MTT assay and a Cell Proliferation Kit I (MTT) (Roche) according to the manufacturer’s protocol. Primary alveolar macrophages were treated with alendronate and cell viability (that is, formation of the insoluble MTT cleavage product) was assessed by dissolving the product in 20% (w/v) SDS and 50% (v/v) dimethylformamide, and the absorbance of the samples at 570 nm was determined using a Denley plate reader. Phagocytosis The effects of alendronate on phagocytosis were investigated in primary alveolar macrophages treated with alendronate for 48 h followed by incubation with 1 mg ml −1 FITC-dextran ( M r =2,000,000; Sigma) at 37 °C for 6 h. The cells were washed three times with PBS. Uptake by macrophages was assessed by dissolving in RPMI 1640, and the absorbance of the samples at 450 nm was determined using a Denley plate reader. Chemotaxis assay The effects of alendronate on the three-dimensional movement of alveolar macrophages were investigated by transwell migration in a Boyden chamber. Primary alveolar macrophages treated with alendronate for 48 h were plated (1 × 10 6 per well) in the upper chamber of Transwells (5-μm pore size polycarbonate membrane; Neuro Probe, Gaithersburg, MD, USA). The cells were incubated at 37 °C for 90 min, rinsed three times with PBS and the cells remaining on top of the polycarbonate membrane were removed. The cells that had migrated through the pores to the lower surface were stained with Diff-Quick. The membranes were mounted on microslides and cells were counted. Western blot analysis Cells were washed twice with PBS, harvested and then lysed in RIPA buffer (20 mM Tris-HCl pH 7.4, 150 mM NaCl, 1% NP-40, 1% Na deoxycholate, 0.1% SDS, deionized water and protease inhibitors). After sonication and removal of debris by centrifugation, 20 μg of protein from each sample was resolved by SDS-polyacrylamide gel electrophoresis and transferred to nitrocellulose membranes. The membranes were immunoblotted with the indicated antibodies: cleaved caspase-3 (1:500), phospho-NF-κB (1:500), NF-κB (1:500), MMP-9 (1:1,000) and β-actin (1:500) and visualized by enhanced chemiluminescence (Amersham Biosciences, Buckinghamshire, England). Enzyme-linked immunosorbent assay The concentrations of TNF-α and IL-1β in the culture medium were measured using a mouse TNF-α enzyme-linked immunosorbent assay (ELISA) kit (R&D Systems, Minneapolis, MN, USA) and IL-1β ELISA kit (R&D Systems), respectively, according to the manufacturer’s instructions. Each sample was assayed in triplicate ( n =5). Cytometric bead array The concentrations of IL-6 and MCP-1 in the culture medium were analysed using Mouse Inflammation Cytometric Beads Array kits (552364, BD Biosciences) according to the manufacturer’s instructions. Analyses were conducted on a FACSCalibur flow cytometer (BD Biosciences). Data were analysed using FCAP Array Software (BD Biosciences). Each sample was assayed in triplicate ( n =5). Statistical analysis Data are expressed as the mean value±s.d.. The significance of differences was examined using Student’s t -test and analysis of variance with Tukey’s post hoc test as appropriate, using SPSS software for Windows. How to cite this article: Ueno, M. et al . Alendronate inhalation ameliorates elastase-induced pulmonary emphysema in mice by induction of apoptosis of alveolar macrophages. Nat. Commun. 6:6332 doi: 10.1038/ncomms7332 (2015).